Mybpc3gene therapy for neonatal cardiomyopathy enables long-term disease prevention in mice Homozygous or compound heterozygous frameshift mutations in MYBPC3 encoding cardiac myosin-binding protein C (cMyBP-C) cause neonatal hypertrophic cardiomyopathy (HCM), which rapidly evolves into systolic heart failure and death within the first year of life. Here we show successful long-term Mybpc3 gene therapy in homozygous Mybpc3 -targeted knock-in (KI) mice, which genetically mimic these human neonatal cardiomyopathies. A single systemic administration of adeno-associated virus (AAV9)- Mybpc3 in 1-day-old KI mice prevents the development of cardiac hypertrophy and dysfunction for the observation period of 34 weeks and increases Mybpc3 messenger RNA (mRNA) and cMyBP-C protein levels in a dose-dependent manner. Importantly, Mybpc3 gene therapy unexpectedly also suppresses accumulation of mutant mRNAs. This study reports the first successful long-term gene therapy of HCM with correction of both haploinsufficiency and production of poison peptides. In the absence of alternative treatment options except heart transplantation, gene therapy could become a realistic treatment option for severe neonatal HCM. Hypertrophic cardiomyopathy (HCM) is the most prevalent inherited cardiac disease with an estimated frequency of 1:500 (ref. 1 ). HCM is transmitted in an autosomal dominant fashion (that is, one affected allele is sufficient to cause disease) and is caused by mutations in genes encoding components of the cardiac sarcomere. Out of them, MYBPC3 encoding cardiac myosin-binding protein C (cMyBP-C) is the most frequently mutated gene. More than 64% of MYBPC3 mutations are truncating, leading to unstable mutant polypeptides [2] , [3] , [4] , [5] . Findings in humans as well as in cat and mouse HCM models indicate that the most prevalent disease mechanism is haploinsufficiency, even for MYBPC3 missense mutations [6] , [7] , [8] . Yet, mutant proteins (‘poison peptides’) may play an additional role in the pathogenesis of the disease [9] , [10] , [11] . HCM is characterized by left ventricular hypertrophy (LVH) with or without left ventricular outflow tract obstruction and consequent congestion, diastolic dysfunction, myocardial disarray and increased interstitial fibrosis. HCM exhibits a large phenotypic variability. Whereas the mean life expectancy of patients who survived into young adulthood does not markedly differ from that of the normal population [12] , sudden cardiac death is common in young adults with HCM, particularly athletes [13] , and some patients develop severe systolic dysfunction and heart failure. Less known is that neonatal forms of HCM rapidly evolve into systolic heart failure and death within the first year of life [14] , [15] , [16] , [17] , [18] , [19] , [20] . Some of these infants have homozygous or compound heterozygous frameshift MYBPC3 mutations [14] , [16] , [17] , [18] , [19] , [20] , expected to result in low level or absence of mutant cMyBP-C. Here we tested the easily generalizable idea to prevent the disease phenotype by adding full-length Mybpc3 by gene therapy in a Mybpc3 -targeted knock-in (KI) mouse model [21] , [22] that genetically mimics the severe neonatal HCM cases [21] , [22] . These mice carry at the homozygous state the human c.772G>A MYBPC3 transition, which is one of the most frequent HCM mutations (13% in a large Italian cohort) [23] and is associated with a bad prognosis [19] . Homozygous KI mice develop systolic dysfunction after postnatal day 1 and LVH at postnatal day 3 (refs 21 , 22 ), but are born with an apparently normal heart, providing the opportunity to treat prior to the onset of the disease phenotype. In the present study, we administered a single dose of adeno-associated virus serotype 9 (AAV9)- Mybpc3 in 1-day-old KI mice. This prevents the development of cardiac hypertrophy and dysfunction and increases Mybpc3 messenger RNA (mRNA) and cMyBP-C protein levels in a dose-dependent manner over a period of 34 weeks (wks). Importantly, Mybpc3 gene therapy also suppresses accumulation of mutant mRNAs. This therapy could be a feasible choice for preventing the development of heart failure and death in neonatal cardiomyopathy. Mybpc3 expression suppresses mutant mRNAs accumulation KI mice carry a G>A transition on the last nucleotide of exon 6, which results in three different mutant mRNAs ( Fig. 1a ) and a >80% reduction of total Mybpc3 mRNA and cMyBP-C protein levels [8] . We first evaluated the level of expression of FLAG-tagged Mybpc3 after gene transfer in cardiac myocytes isolated from KI neonatal mice. Cardiac myocytes were transduced with AAV serotype 6 (AAV6) encoding FLAG-tagged cMyBP-C or green fluorescent protein (GFP) (AAV6- Mybpc3 or AAV6-GFP), under the control of the human cardiac troponin T promoter ( TNNT2 ; Fig. 1b ) for 7 days. Whereas cMyBP-C protein level was low (<20% of wild-type (WT)) in non-transduced or GFP-transduced KI cardiac myocytes, it increased to 70% after AAV6- Mybpc3 gene transfer ( Fig. 2a ). FLAG-cMyBP-C protein was detected in 83% of cMyBP-C-positive cells and was correctly incorporated in doublets in the A-band of the sarcomere ( Fig. 2b ). 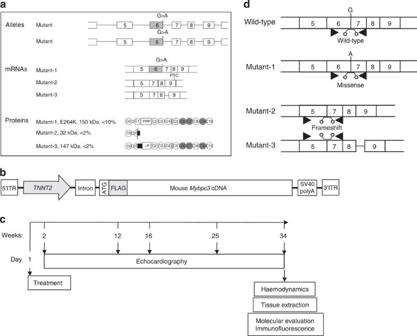Figure 1: Schematic representation of the molecular consequence of the KI mutation, the vector used, protocol forMybpc3gene therapy and location of primers and probes. (a) Consequence of the G>A transition on the last nucleotide ofMybpc3exon 6 at mRNA and protein levels in homozygousMybpc3-targeted knock-in (KI) mice. Mutant-1 mRNA (missense) contains the G>A transition, expected to produce an E264K 150-kDa cMyBP-C. Mutant-2 (nonsense) and mutant-3 (deletion/insertion) mRNAs result from exon-6 skipping. Mutant-2 contains a premature termination codon (PTC) in exon 9 and is expected to produce a 32-kDa truncated cMyBP-C. Mutant-3 mRNA retains parts of intron 8, which restores the reading frame, and should produce a 147-kDa cMyBP-C. (b) Schematic linear representation of the pGG2 vector expressing FLAG-tagged mouse wild-typeMybpc3cDNA under the control of the human cardiac troponin T promoter (TNNT2). (c) Experimental protocolin vivo. Adeno-associated virus serotype 9 (AAV9)-Mybpc3(1 × 1011, 3 × 1011, 1 × 1012or 3 × 1012vector genomes) or PBS was systemically administered in 1-day-old KI mice and compared with wild-type mice. Echocardiography was performed at different postnatal time points until 34 wks of age. At the end of the protocol, mice were subjected to haemodynamics, tissues were extracted and evaluated for molecular biology (RNA and proteins) and for immunofluorescence (cardiac sections). (d) Location of primers (arrows) and Taqman-specific probes (between primers) in wild-type and mutantMybpc3mRNA structures. Figure 1: Schematic representation of the molecular consequence of the KI mutation, the vector used, protocol for Mybpc3 gene therapy and location of primers and probes. ( a ) Consequence of the G>A transition on the last nucleotide of Mybpc3 exon 6 at mRNA and protein levels in homozygous Mybpc3 -targeted knock-in (KI) mice. Mutant-1 mRNA (missense) contains the G>A transition, expected to produce an E264K 150-kDa cMyBP-C. Mutant-2 (nonsense) and mutant-3 (deletion/insertion) mRNAs result from exon-6 skipping. Mutant-2 contains a premature termination codon (PTC) in exon 9 and is expected to produce a 32-kDa truncated cMyBP-C. Mutant-3 mRNA retains parts of intron 8, which restores the reading frame, and should produce a 147-kDa cMyBP-C. ( b ) Schematic linear representation of the pGG2 vector expressing FLAG-tagged mouse wild-type Mybpc3 cDNA under the control of the human cardiac troponin T promoter ( TNNT2 ). ( c ) Experimental protocol in vivo . Adeno-associated virus serotype 9 (AAV9)- Mybpc3 (1 × 10 11 , 3 × 10 11 , 1 × 10 12 or 3 × 10 12 vector genomes) or PBS was systemically administered in 1-day-old KI mice and compared with wild-type mice. Echocardiography was performed at different postnatal time points until 34 wks of age. At the end of the protocol, mice were subjected to haemodynamics, tissues were extracted and evaluated for molecular biology (RNA and proteins) and for immunofluorescence (cardiac sections). ( d ) Location of primers (arrows) and Taqman-specific probes (between primers) in wild-type and mutant Mybpc3 mRNA structures. 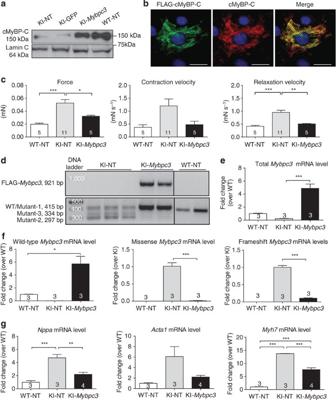Figure 2: Impact ofMybpc3gene transfer in cardiac myocytes in two-dimensional (2D) culture or three-dimensional (3D) engineered heart tissue. Cardiac myocytes were isolated from WT or KI neonatal mice, and were immediately transduced or not with AAV6 encoding FLAG-cMyBP-C or GFP under the control of humanTNNT2promoter at a MOI of 3,000 for 7 days in 2D culture (a,b) or at a MOI of 1,000 for 19 days in 3D engineered heart tissue (c–g). (a) Western blot performed on protein extracts of cardiac myocytes stained with anti-cMyBP-C and anti-lamin A/C antibodies. (b) Immunofluorescence analysis of AAV6-Mybpc3-transduced KI cardiac myocytes. Cells were double-stained with anti-FLAG and anti-cMyBP-C antibodies. Nuclei were stained with DRAQ5. Scale bar, 20 μm. (c) Contractile function of spontaneously beating EHTs measured with video-optical recording. Force, contraction velocity and relaxation velocity were measured at day 19 in culture medium containing 1.8 mM Ca2+. Number of EHTs is indicated in the bars. (d) RT-PCR of exogenous (FLAG-Mybpc3) and totalMybpc3(including WT and/or mutants) mRNAs amplified with specific and common primers, respectively, in RNA fromMybpc3-transduced KI and KI-NT and WT-NT EHTs. Amplicon size is shown on the left side. (e) TotalMybpc3mRNA level determined by RT-qPCR with SYBR Green in RNA from WT-NT, KI-NT and KI-Mybpc3EHTs. (f) Levels of wild-type, missense and frameshift (mutant-2+mutant-3) mRNAs in RNA from WT-NT, KI-NT and KI-Mybpc3EHTs determined with specific hydrolysis Taqman probes. (g) mRNA levels of hypertrophic markers determined by RT-qPCR. All mRNAs were normalized to GαS. Data are expressed as mean±s.e.m. *P<0.05, **P<0.01 and ***P<0.001, one-way ANOVA plus Bonferroni’s post-test (ine,g) or Student’st-test (inf). For mRNA analysis, 3–4 EHTs per group were included. Each qPCR was done in triplicate.Acta1, α-skeletal actin; EHT, engineered heart tissue; KI, knock-in; MOI, multiplicity of infection;Myh7, β-myosin heavy chain;Nppa, atrial natriuretic factor; NT, non-transduced; WT, wild-type. Full size image Figure 2: Impact of Mybpc3 gene transfer in cardiac myocytes in two-dimensional (2D) culture or three-dimensional (3D) engineered heart tissue. Cardiac myocytes were isolated from WT or KI neonatal mice, and were immediately transduced or not with AAV6 encoding FLAG-cMyBP-C or GFP under the control of human TNNT2 promoter at a MOI of 3,000 for 7 days in 2D culture ( a , b ) or at a MOI of 1,000 for 19 days in 3D engineered heart tissue ( c – g ). ( a ) Western blot performed on protein extracts of cardiac myocytes stained with anti-cMyBP-C and anti-lamin A/C antibodies. ( b ) Immunofluorescence analysis of AAV6- Mybpc3 -transduced KI cardiac myocytes. Cells were double-stained with anti-FLAG and anti-cMyBP-C antibodies. Nuclei were stained with DRAQ5. Scale bar, 20 μm. ( c ) Contractile function of spontaneously beating EHTs measured with video-optical recording. Force, contraction velocity and relaxation velocity were measured at day 19 in culture medium containing 1.8 mM Ca 2+ . Number of EHTs is indicated in the bars. ( d ) RT-PCR of exogenous (FLAG- Mybpc3 ) and total Mybpc3 (including WT and/or mutants) mRNAs amplified with specific and common primers, respectively, in RNA from Mybpc3 -transduced KI and KI-NT and WT-NT EHTs. Amplicon size is shown on the left side. ( e ) Total Mybpc3 mRNA level determined by RT-qPCR with SYBR Green in RNA from WT-NT, KI-NT and KI- Mybpc3 EHTs. ( f ) Levels of wild-type, missense and frameshift (mutant-2+mutant-3) mRNAs in RNA from WT-NT, KI-NT and KI- Mybpc3 EHTs determined with specific hydrolysis Taqman probes. ( g ) mRNA levels of hypertrophic markers determined by RT-qPCR. All mRNAs were normalized to GαS. Data are expressed as mean±s.e.m. * P <0.05, ** P <0.01 and *** P <0.001, one-way ANOVA plus Bonferroni’s post-test (in e , g ) or Student’s t -test (in f ). For mRNA analysis, 3–4 EHTs per group were included. Each qPCR was done in triplicate. Acta1 , α-skeletal actin; EHT, engineered heart tissue; KI, knock-in; MOI, multiplicity of infection; Myh7 , β-myosin heavy chain; Nppa , atrial natriuretic factor; NT, non-transduced; WT, wild-type. Full size image We then evaluated whether AAV6- Mybpc3 gene transfer prevented a KI disease phenotype in three-dimensional engineered heart tissue (EHT) generated from neonatal mice. As shown earlier, KI EHTs exhibit higher sensitivity to external Ca 2+ and higher mRNA levels of hypertrophic markers than WT EHTs [24] . As expected, force of contraction and velocity of both contraction and relaxation were higher in non-transduced KI than WT EHTs ( Fig. 2c ) and were not affected by AAV6-GFP. On the other hand, all parameters were lower in AAV6- Mybpc3 -transduced KI EHTs than in non-transduced KI, almost reaching values of non-transduced WT EHTs. This suggests that AAV6- Mybpc3 gene transfer prevented the KI EHTs phenotype (=reduction of hypercontractility). Reverse transcription (RT)-PCR using specific primers ( Supplementary Table 1 ) revealed a FLAG- Mybpc3 mRNA product only in KI EHTs transduced with AAV6- Mybpc3 , but not in the other EHTs ( Fig. 2d ). Analysis of total Mybpc3 mRNA using common primers revealed mutant-1, mutant-2 and mutant-3 mRNAs ( Fig. 1a ) in non-transduced KI EHTs ( Fig. 2d ). In contrast, AAV6- Mybpc3- transduced EHTs exhibited mainly a single mRNA PCR product, similar to WT EHTs ( Fig. 2d ). RT-quantitative (q)PCR with specific Taqman probes ( Fig. 1d ; Supplementary Table 1 ) performed in pooled RNAs confirmed a marked accumulation of WT mRNAs and disappearance of missense (mutant-1) and frameshift (mutant-2 and mutant-3) mRNAs in EHTs transduced with AAV6- Mybpc3 ( Fig. 2e,f ). This suggests that exogenous Mybpc3 expression unexpectedly prevented accumulation of mutant mRNAs in KI EHTs. Moreover, AAV6- Mybpc3 transduction reduced elevated mRNA levels of hypertrophy markers in KI EHTs ( Fig. 2g ). These data suggest that ex vivo Mybpc3 gene therapy prevents both the molecular and functional disease phenotype of KI EHTs. Long-term prevention of LVH and dysfunction by gene therapy Next we evaluated whether Mybpc3 gene therapy could prevent the molecular and functional disease phenotype of KI mice in vivo . KI mice are born without a disease phenotype, but develop reduced fractional area shortening (FAS) between days 1 and 2 and increased left ventricular mass-to-body-weight ratio (LVM/BW) at postnatal days 3–4 (refs 21 , 22 ). Escalating doses of AAV9- Mybpc3 (1 × 10 11 , 3 × 10 11 , 1 × 10 12 and 3 × 10 12 vector genomes (vg)) or phosphate-buffered saline (PBS) were administered into the temporal vein [21] , [22] , [25] of 1-day-old KI mice ( Fig. 1c ). A total of 10 mice per AAV9 dose (except for the 1 × 10 11 dose, n =6) were included in the study ( Supplementary Table 2 ). Some pups treated with AAV9 died during the first weeks, which was independent of the dose administered, but was related to some mothers eating their pups. A total of 5–7 mice treated with AAV9 per group remained and were compared with 12 KI-PBS and 10 WT mice. Cardiac function was evaluated by serial echocardiography at 2, 12, 16, 25 and 34 wks of age ( Fig. 1c ). As expected, PBS-injected KI mice had already an almost two-fold higher LVM/BW ratio at 2 wks of age, which was due to more than two-fold higher LVM despite the 20% higher BW, and 32% lower FAS than WT ( Fig. 3a–d ). BW was higher and independent of the treatments in all KI than WT mice ( Fig. 3b ), indicating that KI mice gained weight quicker than WT mice. AAV9- Mybpc3 prevented the increase in LVM/BW ratio in a dose-dependent manner ( Fig. 3c ). Whereas AAV9 doses of 1 × 10 11 and 3 × 10 11 vg did not have an apparent therapeutic effect, KI mice treated with the highest dose did not differ from WT, but significantly differed from KI-PBS mice. Although the therapeutic effect of Mybpc3 gene therapy on FAS was less marked than that on LVM/BW, there was also a dose-dependent trend towards prevention of cardiac dysfunction at 2 wks of age ( Fig. 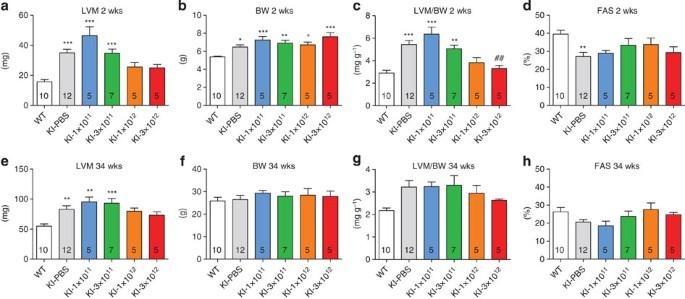Figure 3: Impact of gene therapyin vivo—evaluation of cardiac phenotype by echocardiography. AAV9 (1 × 1011, 3 × 1011, 1 × 1012or 3 × 1012vector genomes) encoding FLAG-cMyBP-C was systemically administered via the temporal vein in 1-day-old KI mice and compared with age-matched PBS-treated KI and WT mice 2 wks (a–d) and 34 wks (e–h) post AAV9 administration. (a,e) Left ventricular mass (LVM). (b,f) Body weight (BW). (c,g) Left ventricular mass-to-body-weight ratio (LVM/BW). (d,h) Fractional area shortening (FAS). Values are mean±s.e.m. *P<0.05, **P<0.01, ***P<0.001 versus WT and##P<0.01 versus KI-PBS, one-way ANOVA plus Bonferroni’s post-test. Number of mice is indicated in the bars. 3d ; Supplementary Table 3 ). Similar results were observed 12, 16 and 25 wks after treatment ( Supplementary Table 3 ). Long-term effect of AAV9- Mybpc3 gene therapy was eventually evaluated 34 wks post administration and exhibited dose-dependent prevention of the increase in LVM/BW and decrease in FAS ( Fig. 3e–h ; Supplementary Table 3 ). Figure 3: Impact of gene therapy in vivo —evaluation of cardiac phenotype by echocardiography. AAV9 (1 × 10 11 , 3 × 10 11 , 1 × 10 12 or 3 × 10 12 vector genomes) encoding FLAG-cMyBP-C was systemically administered via the temporal vein in 1-day-old KI mice and compared with age-matched PBS-treated KI and WT mice 2 wks ( a – d ) and 34 wks ( e – h ) post AAV9 administration. ( a , e ) Left ventricular mass (LVM). ( b , f ) Body weight (BW). ( c , g ) Left ventricular mass-to-body-weight ratio (LVM/BW). ( d , h ) Fractional area shortening (FAS). Values are mean±s.e.m. * P <0.05, ** P <0.01, *** P <0.001 versus WT and ## P <0.01 versus KI-PBS, one-way ANOVA plus Bonferroni’s post-test. Number of mice is indicated in the bars. Full size image To evaluate contractile function with a second method, mice were subjected to haemodynamic measurements by LV catheterization before killing at 34 wks of age ( Figs 1c and 4 ). Some of the mice, independently of the genotype or treatment, could not be analysed due to technical problems (for example, intubation, ventilation or bleeding). Systolic function (d P /d t max ) was slightly, but non-significantly lower in PBS-treated KI than in WT mice ( P <0.06, Student’s t -test; Fig. 4a ). Whereas d P /d t max did not differ between KI-3 × 10 11 vg and KI-PBS, it was higher in KI treated with the two highest doses of AAV9- Mybpc3 than KI-PBS ( P <0.05, Student’s t -test) and did not differ from WT mice ( P =0.6, Student’s t -test; Fig. 4a ). Diastolic function (d P /d t min ) was markedly lower (−44%) in PBS-treated KI, and this reduction was partially prevented in KI mice treated with the two highest doses of AAV9- Mybpc3 ( P =0.02 and 0.07 versus WT, respectively, Student’s t -test; Fig. 4b ). Heart weight (HW) to BW (HW/BW) and HW-to-tibia-length (HW/TL) ratios as measured after killing in all animals were 52–55% higher in PBS-treated KI than in WT mice ( Fig. 4c,d ). Mybpc3 gene therapy induced a dose-dependent reduction in HW/BW and HW/TL ratios, confirming the echocardiographic data with less intra-group variability. The two highest doses groups did not differ from WT. 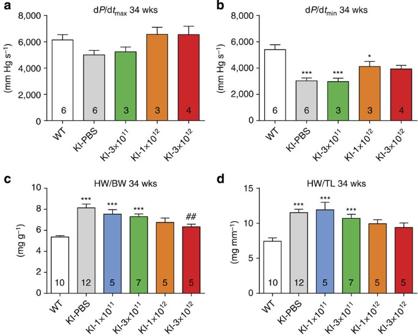Figure 4: Haemodynamic measurements and cardiac hypertrophy determination 34 weeks after AAV9-Mybpc3administration. AAV9-Mybpc3(1 × 1011, 3 × 1011, 1 × 1012or 3 × 1012vector genomes)-treated KI mice were compared with age-matched PBS-treated KI and WT mice. (a) Systolic function (dP/dtmax). (b) Diastolic function (dP/dtmin). (c) Heart weight to body weight ratio (HW/BW). (d) Heart weight to tibia length ratio (HW/TL). Values are mean±s.e.m. *P<0.05 and ***P<0.001 versus WT,##P<0.01 versus KI-PBS, one-way ANOVA plus Bonferroni’s post-test. Number of mice is indicated in the bars. The mice that received 1 × 1011vector genomes were not analysed by haemodynamics. Figure 4: Haemodynamic measurements and cardiac hypertrophy determination 34 weeks after AAV9- Mybpc3 administration. AAV9- Mybpc3 (1 × 10 11 , 3 × 10 11 , 1 × 10 12 or 3 × 10 12 vector genomes)-treated KI mice were compared with age-matched PBS-treated KI and WT mice. ( a ) Systolic function (d P /d t max ). ( b ) Diastolic function (d P /d t min ). ( c ) Heart weight to body weight ratio (HW/BW). ( d ) Heart weight to tibia length ratio (HW/TL). Values are mean±s.e.m. * P <0.05 and *** P <0.001 versus WT, ## P <0.01 versus KI-PBS, one-way ANOVA plus Bonferroni’s post-test. Number of mice is indicated in the bars. The mice that received 1 × 10 11 vector genomes were not analysed by haemodynamics. Full size image To assess the average level of Mybpc3 overexpression, pools of ventricular RNA and proteins were made by combining identical amounts from all 34-wk-old KI and WT mice. Exogenous FLAG- Mybpc3 mRNA was detected only in mice that received AAV9- Mybpc3 , and its level increased with increasing AAV9- Mybpc3 dose ( Fig. 5a ). Mybpc3 gene therapy also dose-dependently increased the level of total full-length Mybpc3 mRNA, and, similar to the effect observed in EHTs, reduced the level of mutant Mybpc3 mRNAs ( Fig. 5a ). At the highest AAV9 dose (=3 × 10 12 vg), mutant Mybpc3 mRNAs were barely detected. Total Mybpc3 mRNA level in KI-PBS mice represented 15% of the WT mouse level ( Fig. 5b ). This level did not differ with the first three AAV9 doses, whereas the highest AAV9- Mybpc3 dose almost fully restored the amount of total Mybpc3 mRNA to the WT level ( Fig. 5b ). The levels of WT and mutant Mybpc3 mRNAs were then determined by RT-qPCR with specific Taqman probes. Whereas WT mRNA level dose-dependently increased in KI up to 64% of the level found in WT mice, missense and frameshift mRNA levels dose-dependently decreased simultaneously ( Fig. 5c ). With the highest AAV9 dose, missense mRNA was fully suppressed and frameshift mRNA decreased by 33%, resulting in the estimation that <6% of total mRNAs is frameshift and the rest is WT. Similar to the mRNA level, the level of exogenous FLAG-cMyBP-C protein increased with increasing AAV9- Mybpc3 doses in pooled proteins ( Fig. 5d ). The level of full-length cMyBP-C protein normalized to glyceraldehyde 3-phosphate dehydrogenase (GAPDH) in AAV9- Mybpc3 -treated KI with the highest dose reached 57% of that in WT mice. These data in pooled samples were supported by statistical analyses of individual samples (=59% of that in WT, Fig. 5e ). 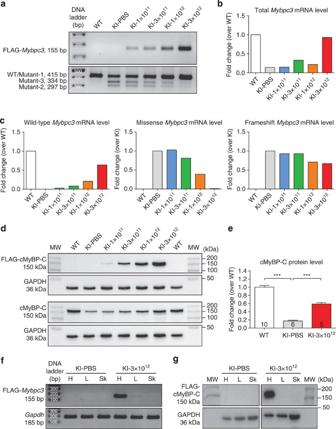Figure 5: Evaluation ofMybpc3expression after AAV9-mediatedMybpc3gene therapyin vivo. Ventricular tissues were extracted from 34-wks-old KI and WT mice that received or not AAV9 (1 × 1011, 3 × 1011, 1 × 1012or 3 × 1012vector genomes) encoding FLAG-cMyBP-C. (a) RT-PCR of exogenous (FLAG-Mybpc3) and totalMybpc3(including WT and/or mutants) mRNAs amplified with specific and common primers in pooled ventricular RNA, respectively (n=5–10 per group). Amplicon sizes are shown on the left side. (b) TotalMybpc3mRNA level determined by RT-qPCR with SYBR Green in pooled ventricular RNA from all groups. (c) Levels of wild-type, missense and frameshift (mutant-2+mutant-3)Mybpc3mRNAs determined with specific hydrolysis Taqman probes in pooled ventricular RNA from all groups. (d) Western blots performed in pooled ventricular protein extracts (n=5–10 per group) were stained with antibodies directed against exogenous FLAG-cMyBP-C, total cMyBP-C or endogenous glyceraldehyde 3-phosphate dehydrogenase (GAPDH). (e) Quantification of cMyBP-C protein level in individual samples from WT, KI-PBS and KI-3 × 1012, normalized to Ponceau and related to WT. (f) RT-PCR of FLAG-Mybpc3andGapdhin heart (H), liver (L), skeletal muscle (Sk) of KI-PBS and KI-3 × 1012mice. MW of the amplicons is shown on the left side. (g) Western blots performed with antibodies directed against exogenous FLAG-cMyBP-C or GAPDH in heart (H), liver (L), skeletal muscle (Sk) of KI-PBS and KI-3 × 1012mice. Values are mean±s.e.m. ***P<0.001, one-way ANOVA plus Dunnett’s post-test versus KI-PBS. Number of mice is indicated in the bars. Each qPCR was performed in triplicate. KI, knock-in; MW, molecular weight markers; WT, wild-type. Figure 5: Evaluation of Mybpc3 expression after AAV9-mediated Mybpc3 gene therapy in vivo . Ventricular tissues were extracted from 34-wks-old KI and WT mice that received or not AAV9 (1 × 10 11 , 3 × 10 11 , 1 × 10 12 or 3 × 10 12 vector genomes) encoding FLAG-cMyBP-C. ( a ) RT-PCR of exogenous (FLAG- Mybpc3 ) and total Mybpc3 (including WT and/or mutants) mRNAs amplified with specific and common primers in pooled ventricular RNA, respectively ( n =5–10 per group). Amplicon sizes are shown on the left side. ( b ) Total Mybpc3 mRNA level determined by RT-qPCR with SYBR Green in pooled ventricular RNA from all groups. ( c ) Levels of wild-type, missense and frameshift (mutant-2+mutant-3) Mybpc3 mRNAs determined with specific hydrolysis Taqman probes in pooled ventricular RNA from all groups. ( d ) Western blots performed in pooled ventricular protein extracts ( n =5–10 per group) were stained with antibodies directed against exogenous FLAG-cMyBP-C, total cMyBP-C or endogenous glyceraldehyde 3-phosphate dehydrogenase (GAPDH). ( e ) Quantification of cMyBP-C protein level in individual samples from WT, KI-PBS and KI-3 × 10 12 , normalized to Ponceau and related to WT. ( f ) RT-PCR of FLAG- Mybpc3 and Gapdh in heart (H), liver (L), skeletal muscle (Sk) of KI-PBS and KI-3 × 10 12 mice. MW of the amplicons is shown on the left side. ( g ) Western blots performed with antibodies directed against exogenous FLAG-cMyBP-C or GAPDH in heart (H), liver (L), skeletal muscle (Sk) of KI-PBS and KI-3 × 10 12 mice. Values are mean±s.e.m. *** P <0.001, one-way ANOVA plus Dunnett’s post-test versus KI-PBS. Number of mice is indicated in the bars. Each qPCR was performed in triplicate. KI, knock-in; MW, molecular weight markers; WT, wild-type. Full size image To assess whether AAV9-mediated gene therapy with a cardiac-specific promoter carries the risk of off-target effects in other organs, we took tissue samples from liver and skeletal muscle of one of the AAV9- Mybpc3 -treated KI mice treated with the highest dose and subjected them to RT-PCR and western blot. FLAG- Mybpc3 mRNA was amplified in ventricles, and to a very low extent in liver or skeletal muscle ( Fig. 5f ). FLAG-cMyBP-C protein was only detected in the ventricles, but not in liver and skeletal muscle ( Fig. 5g ). Evaluation of cardiac sections by immunofluorescence showed exogenous FLAG-cMyBP-C protein to be organized in doublets in the A-band of the sarcomere and in alternation with α-actinin, indicating correct sarcomeric incorporation ( Fig. 6a ). Of note, not all α-actinin-positive cardiac myocytes were FLAG-positive, suggesting incomplete transduction. A cMyBP-C antibody recognizing both endogenous and exogenous cMyBP-C proteins showed typical A-band doublets throughout the section in WT mice and a much weaker, less-defined signal in PBS-treated KI, reflecting the lower total cMyBP-C protein amount in KI ( Fig. 6b ). The signal was much stronger in AAV9- Mybpc3 -treated KI, but again, not all cardiac myocytes were stained. 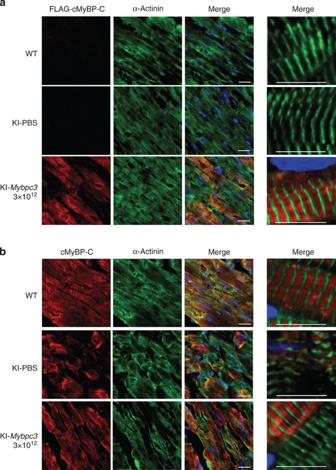Figure 6: Immunofluorescence analysis of cardiac sections 34 weeks after AAV9-Mybpc3administration. Hearts from WT, KI treated with PBS or with 3 × 1012virus genomes of AAV9-Mybpc3were extracted and cryosections were performed. (a) Double-staining of cardiac sections with anti-FLAG and anti-α-actinin antibodies. (b) Double-staining of cardiac sections with anti-cMyBP-C and anti-α-actinin antibodies. Nuclei were stained with DRAQ5. Scale bar, 20 μm. Merge images on the right panel were obtained at a higher magnification (scale bar, 10 μm). Figure 6: Immunofluorescence analysis of cardiac sections 34 weeks after AAV9- Mybpc3 administration. Hearts from WT, KI treated with PBS or with 3 × 10 12 virus genomes of AAV9- Mybpc3 were extracted and cryosections were performed. ( a ) Double-staining of cardiac sections with anti-FLAG and anti-α-actinin antibodies. ( b ) Double-staining of cardiac sections with anti-cMyBP-C and anti-α-actinin antibodies. Nuclei were stained with DRAQ5. Scale bar, 20 μm. Merge images on the right panel were obtained at a higher magnification (scale bar, 10 μm). Full size image This study reports the first successful long-term gene therapy of HCM, the most common inherited cardiac disease. Several aspects are notable: (i) AAV-mediated Mybpc3 expression not only corrected the reduction of total cMyBP-C mRNA and protein levels as expected, but also suppressed the production of mutant mRNA species, which may give rise to pathological proteins. Thus, Mybpc3 gene therapy appears to correct both haploinsufficiency and poison peptide mechanisms as underlying causes of HCM. (ii) In fact, our Mybpc3 gene therapy approach was functionally successful in a KI mouse model of HCM, which exhibits both the reduction of total mRNA/protein levels and pathological mRNA species. (iii) The prevention of the disease phenotype by gene therapy was clearly AAV9-dose-dependent, almost complete and long lasting. (iv) By principle, Mybpc3 gene therapy, in contrast to mutation-specific therapy approaches, should be applicable to all forms of HCM caused by MYBPC3 gene mutations. Thus, the present data are an important step towards clinical translation of gene therapy for patients with severe, MYBPC3 -related forms of HCM. Gene therapy for HCM comes in the continuity of gene therapy for heart failure, targeting proteins involved in calcium-handling such as phospholamban [26] and S100A1 (ref. 27 ). The recent successful completion of phase II trials of SERCA2a gene therapy demonstrated the feasibility and safety of AAV1-mediated gene transfer as well as improvement of the symptoms and exercise capacity of patients with advanced heart failure [28] . Classical treatments of HCM target symptoms and LV outflow tract obstruction with pharmacological and/or surgical treatments, but do not address the cause of the disease [29] , [30] . New strategies targeting the endogenous mutant pre-mRNA or RNA such as exon skipping, exon inclusion, trans -splicing and RNA silencing, opened the perspective for a causal therapy for patients with HCM [2] , [21] , [22] , [31] , [32] . These proof-of-concept studies still have major limitations. We previously showed that a 5′- trans -splicing approach corrects the mutation in cardiac myocytes and in vivo in HCM KI mice, but its efficiency was too low to prevent or rescue the disease phenotype [22] . In-frame skipping of mutated exons by antisense oligonucleotides inserted in U7snRNA produced a stable functional protein and transiently rescued the cardiac phenotype in KI mice [21] . In both cases, however, the amount of repaired protein remained very low [21] , [22] . Another RNA-targeting approach, the allele-specific silencing using oligonucleotides has been recently evaluated in another HCM mouse model carrying a mutation in Myh6 encoding α-myosin heavy chain showing disease prevention until 25 wks of age, which, in this model, needs to be revealed by application of cyclosporine [31] . The present Mybpc3 gene therapy approach was not a priori considered as a feasible therapy strategy for HCM for two reasons. First, it is generally assumed that the packaging capacity of AAV is limited to ~4.9 kbp, while longer sequences have been shown to lead to truncation of AAV particles [33] or to markedly decrease transduction efficiency [34] . However, we demonstrate herein that packaging of an oversized DNA sequence of 5.4 kbp (including two inverted terminal repeats, the human TNNT2 promoter, a chimeric intron, the FLAG-tagged Mybpc3 complementary DNA (cDNA) and the SV40 polyadenylation signal) was compatible with efficient production of AAV6 and AAV9, and that the vectors induced efficient expression of full-length Mybpc3 in isolated mouse cardiac myocytes and EHTs, as well as in the mouse heart in vivo . Second, it was not expected that expression of the WT protein also prevents the production of mutant mRNAs. Yet, this was the case both ex vivo and in vivo , and this was dose-dependent. The molecular mechanism is not clear at present, but the paracrystalline structure of sarcomeric scaffolding suggests that sarcomeric proteins, in particular those contributing to the contractile mechanism such as actins and myosins, are in a precise stoichiometric equilibrium [35] . As AAV-induced WT cMyBP-C protein would be more stably integrated into the sarcomere, yet unknown feedback mechanisms might downregulate transcription of the mutant allele. If this hypothesis was true, gene therapy could be principally used for other dominant sarcomeric gene mutations since the stoichiometry of the sarcomere should be conserved. Whereas the latter idea needs experimental confirmation, the observed suppression of pathologic mRNA species by gene therapy is clearly important. Indeed, we previously showed that, in contrast to homozygous knockout mice that are deficient in cMyBP-C, the presence of even a low level of cMyBP-C mutants in homozygous and heterozygous KI mice have a dominant-negative effect on the function of the ubiquitin–proteasome system upon adrenergic stress or aging [9] , [10] , [11] . Long-term expression of cMyBP-C in the heart was achieved by a single intravenous injection in 1-day-old KI mice using a combination of AAV9, which is the most cardiotropic serotype in rodents [21] , [36] and a cardiomyocyte-specific promoter [36] , [37] . Previous data indicated that combining AAV9 and a chicken minimal truncated TNNT2 promoter gave >640-fold higher expression in the heart than in other organs in mice [37] . Here, we used a human minimal truncated TNNT2 promoter that showed restriction of FLAG-cMyBP-C protein expression to the heart 34 wks following systemic administration in vivo , supporting recent data using the same combination of AAV9 and TNNT2 promoter 13 wks after injection [38] . Serial echocardiographic analyses were done by a highly experienced investigator blinded to the genotype or treatment group. It still showed relevant intra- and inter-subject variability over time and, due to multiple group testing (two-way analysis of variance (ANOVA) for groups and time points) and the relatively small number of mice in each group ( n =5–12), only reached significant differences between PBS-treated KI and WT. However, separated evaluation at all time points using one-way ANOVA showed significant difference between groups with respect to different parameters, including LVM/BW and FAS ( Supplementary Table 3 ). In addition, HW/BW and HW/TL ratios, very robust parameters, revealed clear and significant effects of gene therapy. Furthermore, the dose dependency of the functional improvement and the haemodynamic data all support the conclusion that gene therapy in newborn KI mice partially prevented the disease phenotype. Of note, the effect of Mybpc3 gene therapy was larger than anything reported previously [21] , [22] , but still remained incomplete, both in terms of molecular and functional restoration. Whereas total Mybpc3 mRNA levels almost reached WT levels in KI treated with the highest dose, protein levels reached maximally ~60% of WT levels. This incomplete restoration is also revealed by the patchy pattern as shown by immunofluorescence, that is, some cells showed normal staining, others no staining at all. Likely, the WT protein level per ventricular myocytes cannot exceed 100%, whereas mRNA levels can [35] , resulting in slightly different average mRNA and protein levels after gene transfer. In addition, the stability of the exogenous protein could be slightly altered (reduced translation or accelerated degradation). Finally, some cardiac myocytes may undergo cell division after birth and therefore loose the AAV9 (ref. 39 ). Limitations of the study should be noted. First, it showed prevention of a disease phenotype, but no rescue. Yet, we believe that prevention is the more realistic scenario in the patient group we would like to target with the gene therapy approach, namely infants with severe homozygous or compound heterozygous mutations who quickly develop a therapy-resistant form of systolic heart failure [14] , [16] , [17] , [18] , [19] , [20] . Second, mouse models including our KI model clearly differ from human HCM in that they show a much milder phenotype, generally only at the homozygous state [8] , [40] , [41] . In fact, our KI mice, although likely the best murine HCM model available, have a normal life expectancy and, as shown also in this study, LVH and the decrease in LV contractile function remain stable over time. However, this also means that the maximal therapeutic effect is smaller than expected for large animals or humans with homozygous mutations. Finally, practical issues such as the presence of neutralizing antibodies against AAV9 do not need to be considered in mice, but may constitute a real problem in patients particularly in infants [42] . In summary, the present study reports the first successful long-term gene therapy of HCM that should be principally applicable to all forms of severe HCM caused by mutations in MYBPC3 . The target population for such therapy are newborn children with homozygous or compound heterozygous MYBPC3 mutations who, similar to KI mice, are born relatively normal, but quickly develop severe LV dysfunction and dyspnoea, dying on average within 1 year. We believe that for such children MYBPC3 gene therapy could be a realistic option and we currently work on translating the concept to a large animal model. Animals The investigation conforms to the guidelines for the care and use of laboratory animals published by the NIH (Publication No. 85–23, revised 1985). The experimental procedures were in accordance with the German Law for the Protection of Animals and accepted by the Ministry of Science and Public Health of the City State of Hamburg, Germany (No. 69/10). KI mice were generated previously [8] , and both KI and WT mice were maintained on a Black Swiss background. FLAG- Mybpc3 construct The pGG2- TNNT2 -FLAG- Mybpc3 was generated by an exchange of the cytomegalovirus-intron cassette of the pGG2 expression vector with the TNNT2 -intron cassette derived from the shuttle plasmid pds- TNNT2 -Rluc by double digestion with EcoRI/NheI. The full-length FLAG- Mybpc3 cDNA comprising exons 1–34 was amplified by PCR from murine ventricular WT Mybpc3 cDNA with the forward primer including the XhoI restriction site, the ATG followed by the FLAG sequence and the first 20 nt of Mybpc3 exon 1. The reverse primer contained the last 4 nucleotides of exon 33 plus 8 nucleotides of exon 34, the TGA stop codon followed by the BamHI restriction site. The PCR was done using a touchdown program (70 °C–65 °C) with Phusion Hot Start II High-Fidelity DNA polymerase and 36 cycles. PCR product and the pGG2- TNNT2 vector were then XhoI/BamHI digested and purified by gel extraction. After ligation, ampicillin-resistant clones were tested by enzymatic digestion for presence of the insert and one positive pGG2- TNNT2 -FLAG- Mybpc3 clone was sequenced. Production and titration of AAV particles AAV6 pseudotyped vectors were generated by co-transfection of HEK293-AAV cells (Biocat) with the pdsAAV- TNNT2- FLAG- Mybpc3 transfer plasmid and the AAV-packaging plasmid pDP6rs, which provides the AAV2 rep and AAV6 cap genes and adenoviral helper functions. AAV9 pseudotyped vectors were generated by triple-transfection of pdsAAV -TNNT2 -FLAG- Mybpc3 transfer plasmid with pAAV2/9 and pHelper encoding adenoviral helper functions (Biocat). Generation of recombinant AAV6 and AAV9 particles was carried out as follow. Briefly, 1.5 × 10 7 HEK293-AAV cells were seeded on 15-cm plates and transfected with polyethylenimine. Three days after transfection cells were collected, washed three times with PBS and resuspended in PBS. Three cycles of freeze–thaw were done before incubation (1 h at 37 °C) with benzonase (Merk; final concentration 250 U ml −1 ). Cells debris were pelleted and vector-containing lysate were purified by iodixanol step gradients. The genomic titres of AAV6 and AAV9 were determined by qPCR using SYBR Green qPCR Master Mix2 (Fermentas) and an ABI PRISM 7900HT cycler (Applied Biosystem). Vectors were titrated using primers specific for the TNNT2 promoter sequence and a standard curve obtained by serial dilutions of the respective plasmids. Experiments in neonatal mouse cardiac myocytes Neonatal mouse cardiac myocytes (NMCMs) were isolated from at least 20 hearts of 1–4-day-old KI mice after an overnight incubation with 0.5 mg ml −1 trypsin followed by repeated digestion with 240 U ml −1 collagenase type II. The isolated cells were then pre-plated twice to exclude non-muscle cells. NMCMs were finally plated on laminin-coated dishes at a density of 10 5 cells cm −2 . AAV6-mediated transductions of cardiac myocytes were performed for 30 min at 37 °C in suspension prior to plating (4.4 × 10 5 cells per well) at a multiplicity of infection of 3,000. Cardiac myocytes were kept in culture for 7 days at 37 °C and 10% CO 2 prior to collection. Experiments in mouse EHTs EHTs were generated from unpurified mouse cardiac cells [24] . In brief, isolated cells were resuspended at a density of 6.8 × 10 6 cells ml −1 in culture medium containing bovine fibrinogen (5 mg ml −1 ), aprotinin (2.5 μg ml −1 ) and 10% Matrigel (BD Bioscience). The reconstitution mix (97 μl/EHT) was mixed with thrombin (3 μl/EHT, 100 U ml −1 ) and pipetted into rectangular agarose casting moulds in a 24-well plate. Prior to this pipetting step, silicon racks with four pairs of elastic silicone posts each were placed onto the 24-well plate so that one pair of posts reached from the top the cell–fibrinogen–thrombin mix contained in the casting mould. Fibrin polymerization led to a muscle strip around the silicone posts. The racks were then transferred to fresh 24-well plates containing culture medium (Dulbecco’s modified Eagle’s medium, 10% horse serum, 2% chick embryo extract, 1% penicillin/streptomycin, 10 μg ml −1 insulin and 33 μg ml −1 aprotinin) and maintained at 21% oxygen. On day 5 cytosine β- D -arabinofuranoside (25 μg ml −1 ) was added to the culture medium for 48 h. AAV6 transduction (multiplicity of infection 1,000) was performed directly into the freshly isolated heart cells before adding reconstitution mix components and casting EHTs [43] , [44] . Contractility measurements were performed on day 19. Briefly, contractions were measured by video-optical recording using a customized software ( http://www.ctmv.de ), based on figure recognition of the contracting muscle strip in a fully automated manner. Values for average force, contraction and relaxation velocity were calculated with a specific custom-made algorithm. In vivo AAV9 administration One-day-old KI mice received different doses of AAV9 (from 1 × 10 11 to 3 × 10 12 vg per mouse) or PBS via systemic administration into the temporal vein using a 30-G needle [21] , [22] . Echocardiographic analysis Transthoracic echocardiography was performed using the Vevo 2100 System (VisualSonics, Toronto, Canada). Mice were anaesthetized with isoflurane (1–2%) and taped to a warming platform in a supine position. B-mode images were obtained using a MS400 transducer for adult mice and a MS550 transducer for neonatal mice. Images were obtained in a parasternal short and long-axis view and dimensions of the left ventricle were measured in a short-axis view in diastole and systole. In vivo haemodynamics Haemodynamic measurements were performed in an open-chest approach in 34-wk-old mice. Mice were anaesthetized with isoflurane (3.5% for induction, 2% during the recording), and buprenorphine (0.5 mg kg −1 BW) was administered for analgesia. Animals were assured to a warming platform in a supine position. Tracheotomy was performed and mice were artificially ventilated with a rodent ventilator (MiniVent Type 845, Hugo Sachs). The abdomen was opened subxiphoidally. The diaphragm was incised via a transversal subcostal approach and the pericardium was opened. The LV was entered via an apical stab with a 25-gauge needle, followed by a 1.2-F transonic catheter. After a stabilization period of 5 min heart rate, left ventricular end-diastolic and end-systolic pressure and LV systolic (d P /d t max ) and diastolic (d P /d t min ) functions were recorded with the Scisense ADVANTAGE System. RT-PCR and RT-qPCR Total RNA was isolated from ventricular tissue or EHTs using the SV Total RNA Isolation System Kit (Promega) or Trizol reagent, respectively, according to the manufacturer’s instructions. RT was performed from 200 ng RNA from EHTs or pooled RNA (200 ng RNA per sample) using oligo(dT) primers and the SuperScript III kit (Life Technologies). RT-PCR and RT-qPCR were performed with different primer pairs and probes ( Supplementary Table 1 ). Touchdown RT-PCR amplifications (65–60 °C or 60–55 °C depending on primer pairs) were performed using AmpliTaq Gold Polymerase (Applied Biosystem) in a total volume of 20 μl and 35 cycles. PCR products were visualized on 2% agarose gel. RT-qPCR for total Mybpc3 mRNA level and hypertrophic markers were performed with SYBR Green qPCR Master Mix 2 (Fermentas). WT and mutant Mybpc3 mRNA levels were determined with specific hydrolysing probes. Data were normalized to GαS. Western blot analysis For western blots analysis crude proteins were extracted from cultured cardiac myocytes or tissues, separated on 10% SDS-polyacrylamide (29:1) mini-gels (Bio-Rad) and electrotransferred on polyvinylidene difluoride or nitrocellulose membranes. Primary antibodies were directed against the FLAG epitope (1:5,000; Sigma), the MyBP-C motif (1:1,000), lamin A/C (1:2,000; Santa Cruz), or GAPDH (1:2,000; HyTest). Secondary antibodies were anti-mouse (1:20,000; Dianova) or anti-rabbit (1:6,000; Sigma) peroxidase-conjugated. Proteins were visualized using the Super Signal West Dura detection reagent (Thermo Scientific) and signals were detected with the ChemiGenius 2 Bio Imaging System. Full western blots from tissue samples are displayed in Supplementary Fig. 1 . Immunofluorescence analysis For immunofluorescence analysis, AAV6-transduced KI NMCMs were cultured 7 days on glass coverslips prior to fixation with methanol/acetone (20/80) at −20 °C. For immunofluorescence of 10-μm-thick cardiac sections, hearts were rinsed in KCl solution and embedded in Tissue Tek®. After permeabilization, cells and cardiac sections were stained with primary antibodies, the anti-FLAG (1:800, Sigma), anti-cMyBP-C directed against the MyBP-C motif (1:500) and anti-α-actinin (1:800, Sigma). Secondary antibodies were the anti-mouse IgG Alexa 488-conjugated, 1:800 and anti-rabbit IgG Alexa 546-conjugated, 1:800 (Molecular Probes). Nuclei were stained with DRAQ5 (1:1,000; Biostatus). Confocal images were acquired with a Zeiss LSM 710 system using a Zeiss Axiovert microscope. Statistical analysis Data were expressed as mean±s.e.m. Statistical analyses were performed by one-way or two-way ANOVA followed by Dunnett’s or Bonferroni’s post-test, and by the Student’s t -test as indicated in figure legends or text, using the commercial software GraphPad Prism5 (Software Inc.). A value of P <0.05 was considered statistically significant. How to cite this article: Mearini, G. et al. Mybpc3 gene therapy for neonatal cardiomyopathy enables long-term disease prevention in mice. Nat. Commun. 5:5515 doi: 10.1038/ncomms6515 (2014).